Orbitofrontal neurons infer the value and identity of predicted outcomes The best way to respond flexibly to changes in the environment is to anticipate them. Such anticipation often benefits us if we can infer that a change has occurred, before we have actually experienced the effects of that change. Here we test for neural correlates of this process by recording single-unit activity in the orbitofrontal cortex in rats performing a choice task in which the available rewards changed across blocks of trials. Consistent with the proposal that orbitofrontal cortex signals inferred information, firing changes at the start of each new block as if predicting the not-yet-experienced reward. This change occurs whether the new reward is different in number of drops, requiring signalling of a new value, or in flavour, requiring signalling of a new sensory feature. These results show that orbitofrontal neurons provide a behaviourally relevant signal that reflects inferences about both value-relevant and value-neutral information about impending outcomes. The best way to respond flexibly to changes in the environment is to anticipate them. In many cases, such anticipation requires us to infer that a change has occurred, before we have actually experienced the effects of that change. For example, suppose you see your boss striding into his office in the morning with a dark scowl on his face. You realize that he is in a bad mood, and consequently you can change your expectations for what he might say to you in your morning meeting. Note that because you are using inference, the sensory cue—the scowl—need not ever be directly associated with the changed value of his words. But you, having observed the hidden sign and made the inference, can anticipate what will happen next. The orbitofrontal cortex (OFC) has been hypothesized to track such inferred states and to signal information about expected outcomes based on them [1] , [2] , [3] . Indeed, numerous studies have found that neural activity in OFC anticipates expected outcomes [4] , [5] , [6] , [7] , [8] , [9] , [10] , [11] , [12] . However, the question of what function this activity performs has not been fully answered. One idea is that anticipatory activity drives decision making by representing the expected or even economic value of the outcomes that are likely to ensue in a given situation [6] , [13] . However, most OFC neurons track specific features of outcomes, like flavour, or even their context, rather than value, and respond more generally to other events in the environment [6] , [11] , [14] , [15] , [16] , [17] . Furthermore, causal studies have reported that OFC manipulations disrupt value-guided decisions when they are based on inferences and not when they are based on simple comparisons of previously learned values [13] , [18] , [19] , [20] , [21] , [22] , [23] . Here we sought to test for neural correlates of this inferential process by recording single-unit activity in OFC in rats performing a choice task in which, on each trial, the rats chose between two milk rewards, which varied across blocks of trials both in number of drops and flavour. We were specifically interested in how OFC neurons would change firing in anticipation of new rewards at block switches, before those rewards were actually experienced. Consistent with the proposal that OFC infers information about expected outcomes, firing in OFC changed at the start of each new block as if predicting the not-yet-experienced reward. This change predicted the speed of with which choice behaviour was adjusted in that block, and it occurred whether the new reward was different in number of drops, requiring signalling of a new value, or in flavour, requiring signalling of a new sensory feature. These results show that OFC neurons infer both value-relevant and value-neutral information about impending outcomes. Rats ( n =6) were trained in an odour-guided choice task (illustrated in Fig. 1a ) to respond at either a left or right well to receive a small (one drop) or a large (three drops) amount of chocolate or vanilla-flavoured milk. This task was similar to an odour-guided choice task that we have used previously [14] , except that we manipulated reward flavour in some blocks instead of reward delay. Importantly, we used amounts and concentrations that we established separately were equivalently preferred (see Fig. 1b ). Response-reward contingencies were stable across blocks of ~60 trials, but switched unpredictably in reward number or reward flavour at block transitions. Contingencies were arranged so that (i) rewards in the two directions always differed in both number and flavour (for example, large chocolate versus small vanilla or large vanilla versus small chocolate), and (ii) number and flavour switches alternated according to the sequence number-flavour-number-flavour across the five blocks of every session. Free-choice and forced-choice trials, instructed by an odour delivered at the beginning of the trial, were intermixed within blocks but always had the same response-reward contingencies. 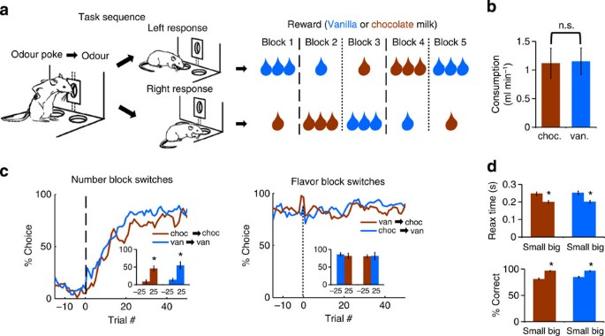Figure 1: Task and behavior. (a) After initiating a trial with a nosepoke, an odour was delivered for 500 ms, after which rats responded at one of the two fluid wells for one or three drops of chocolate (choc.) or vanilla (van.) milk, delivered 500 ms after the well poke. Two odours indicatedforced choices, left or right; a third odour indicatedfree choice.Reward contingencies were stable across blocks of ~60 trials, but switched in number of drops (dashed lines) or flavour (dotted lines) in four unsignalled transitions. Rewards in the two directions always differed in both number of drops and flavour (one of the four possible block sequences is shown). (b) Choc. and van. milk were equally preferred in a 10-min consumption test in a separate group of rats (t10=0.1,P=0.93). (c) Choice rates in the task reflected the number of drops but not the flavour. Number switches (left panel) had a similarly large effect on choice rates for choc.->choc. and van.->van. switches. Flavour switches (right panel) had no effect on choice rates across big van.->big choc. or big choc.->big van. Line figures show average trial-by-trial choice rates; inset bar graphs show choice rates before versus after switches (25 trials each). ANOVA on difference in choice rates across transitions, factors transition type and initial flavour; main effect of transition type (F1,92=195.7,P<0.001), driven by significant changes across number transitions (planned contrast, F1,92=445.9,P<0.0001), and insignificant changes across flavour transitions (planned contrast, F1,92=1.3,P=0.27); no effect of initial flavour (F1,92=0.0,P=0.93); no differences between van.-to-choc. and choc.-to-van. (planned contrast. F1,92=2.3,P=0.13). (d) Reaction time (top panel) and accuracy (bottom panel) reflected the number of drops expected but not the flavour. Bar graphs show average reaction time (from end of odour to movement) or accuracy on forced-choice trials within the last 25 trials of blocks. Within-subjects ANOVAs on reaction time and accuracy: main effects of number (F1,93=62.2,P<0.001; F1,93=182.3,P<0.001) but not flavour (F1,93=0.3,P=0.57; F1,93=5.3,P=0.024†), nor interactions (F1,93=0.1,P=0.73; F1,93=5.1,P=0.027†). Error bars show standard errors; *P<0.001, main effects of number; not significant ifP-value criterion is corrected for the three separate ANOVAs testing flavour effects (P<0.0167 by Bonferroni correction). Figure 1: Task and behavior. ( a ) After initiating a trial with a nosepoke, an odour was delivered for 500 ms, after which rats responded at one of the two fluid wells for one or three drops of chocolate (choc.) or vanilla (van.) milk, delivered 500 ms after the well poke. Two odours indicated forced choices , left or right; a third odour indicated free choice. Reward contingencies were stable across blocks of ~60 trials, but switched in number of drops (dashed lines) or flavour (dotted lines) in four unsignalled transitions. Rewards in the two directions always differed in both number of drops and flavour (one of the four possible block sequences is shown). ( b ) Choc. and van. milk were equally preferred in a 10-min consumption test in a separate group of rats ( t 10 =0.1, P =0.93). ( c ) Choice rates in the task reflected the number of drops but not the flavour. Number switches (left panel) had a similarly large effect on choice rates for choc.->choc. and van.->van. switches. Flavour switches (right panel) had no effect on choice rates across big van.->big choc. or big choc.->big van. Line figures show average trial-by-trial choice rates; inset bar graphs show choice rates before versus after switches (25 trials each). ANOVA on difference in choice rates across transitions, factors transition type and initial flavour; main effect of transition type (F 1,92 =195.7, P <0.001), driven by significant changes across number transitions (planned contrast, F 1,92 =445.9, P <0.0001), and insignificant changes across flavour transitions (planned contrast, F 1,92 =1.3, P =0.27); no effect of initial flavour (F 1,92 =0.0, P =0.93); no differences between van.-to-choc. and choc.-to-van. (planned contrast. F 1,92 =2.3, P =0.13). ( d ) Reaction time (top panel) and accuracy (bottom panel) reflected the number of drops expected but not the flavour. Bar graphs show average reaction time (from end of odour to movement) or accuracy on forced-choice trials within the last 25 trials of blocks. Within-subjects ANOVAs on reaction time and accuracy: main effects of number (F 1,93 =62.2, P <0.001; F 1,93 =182.3, P <0.001) but not flavour (F 1,93 =0.3, P =0.57; F 1,93 =5.3, P =0.024 † ), nor interactions (F 1,93 =0.1, P =0.73; F 1,93 =5.1, P =0.027 † ). Error bars show standard errors; * P <0.001, main effects of number; not significant if P -value criterion is corrected for the three separate ANOVAs testing flavour effects ( P <0.0167 by Bonferroni correction). Full size image The purpose of this task was to compare neural activity after switches in the number of reward drops, in which the value of choices changed, with that after switches in reward flavour, in which there was no change in the value of the two choices. In accord with this distinction, as shown in Fig. 1c , number switches resulted in a fast-developing and sustained change in choice rate on free-choice trials, so that after ~38 trials rats were choosing the side with three drops of milk on ~80% of free-choice trials. The rate with which they made this switch was independent of flavour, and flavour transitions (chocolate to vanilla or vanilla to chocolate) caused no enduring change in choice rate (see figure captions for all statistics). We also examined how reaction time and accuracy on forced-choice trials were influenced by shifts in reward number and flavour. As shown in Fig. 1c,d , reaction time, defined as the time from odour offset to odour port exit, was faster and forced-choice performance was more accurate when a large reward could be expected compared with when a small reward could be expected. Again these effects were independent of reward flavour. Thus, rats’ performance in this task on both free- and forced-choice trials was sensitive to the number of reward drops, thereby reflecting the higher value of a large reward, but insensitive in to their flavour, reflecting the similar value placed on the chocolate and vanilla flavours. We recorded 831 single-units from OFC in six rats during these 94 behavioural sessions, which included all recording sessions in which all five block were completed. The six rats completed 3, 24, 25, 28, 5 and 9 sessions, in which we recorded 28, 170, 275, 246, 28 and 84 single-units, respectively (some rats had fewer than ten completed sessions because of broken electrodes or other technical problems). The locations of the recordings are shown in Fig. 2a . We were interested in reward-anticipatory activity; such activity has been reported frequently in OFC. Thus, we analysed activity in a 500 ms epoch as rats waited in the fluid port, immediately before the first drop of reward was delivered. We performed an analysis of variance (ANOVA) on firing rate for each unit during this epoch with factors reward number, reward flavour and reward location (left or right). We used forced-choice trials for this analysis, because they were equally distributed across the levels of these factors. Many neurons were selective for number or flavour during this epoch ( Fig. 2b–f ). Counting main effects of number along with number × flavour and number × location interactions, 278 neurons (33%) were number anticipatory and 198 (24%) were flavour anticipatory, including 124 (15%) with effects of both number and flavour or interactions between them. In addition, as has been reported previously, many neurons fired selectively in anticipation of rewards according to their location (384, or 46%, showed some effect of reward location), and the majority of neurons with effects of number or flavour also had some effect of location (173 of the 278 neurons with number effects, or 62%, also had location effects; 123 of 198 neurons with flavour effects, or 62%, also had location effects). 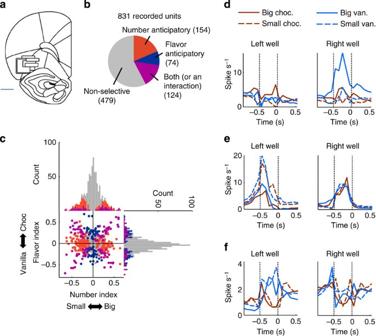Figure 2: Recording sites and characterization of reward-selective activity. (a) The black boxes indicate the approximate location from which recordings were made in each rat (in the left hemisphere). The width represents the estimated span of the electrode bundle (~1 mm), and the height represents the approximate extent of recording across all sessions. Bregma +2.8 to 3.6 mm; scale bar=1 mm. (b) The coloured sections represent the proportion of the entire population with significant effects of number of drops, flavour or both, based on a three-way ANOVA performed on firing rate across trials, with factors flavour, number and reward location. The epoch tested was the 500 ms immediately preceding delivery of the first drop of reward. (c) Reward-selective neurons were distributed equally between chocolate (choc.)- and vanilla (van.)-preferring, and between big- and small-preferring. Shown are flavour- and number-selectivity indices calculated for each recorded neuron, colour-coded as inb. The proportions of significant neurons were not significantly different between small versus big or between choc. versus van. byχ2test. Big-preferring, 126 neurons; small-preferring, 152 neurons (χ2stat: 2.4,P=0.12); choc.-preferring, 103 neurons; van.-preferring, 95 neurons (χ2stat: 0.3,P=0.57). Average magnitude of number index for large-preferring versus small-preferring (t276=−1.2,P=0.24); average magnitude of flavour index for choc.-preferring versus van.-preferring (t196=1.1,P=0.29). (d–f) Each plot shows, for a single-unit example, average firing rate for each of the four number/flavour combinations, separately for the left and right wells and aligned on initial reward delivery (at 0 s). Vertical dotted lines show epoch from well-entry to reward delivery. (d) An example with number/flavour interaction, (e) an example with only a number effect and (f) an example with only a flavour effect. All examples shown here have strong effects of location. Figure 2: Recording sites and characterization of reward-selective activity. ( a ) The black boxes indicate the approximate location from which recordings were made in each rat (in the left hemisphere). The width represents the estimated span of the electrode bundle (~1 mm), and the height represents the approximate extent of recording across all sessions. Bregma +2.8 to 3.6 mm; scale bar=1 mm. ( b ) The coloured sections represent the proportion of the entire population with significant effects of number of drops, flavour or both, based on a three-way ANOVA performed on firing rate across trials, with factors flavour, number and reward location. The epoch tested was the 500 ms immediately preceding delivery of the first drop of reward. ( c ) Reward-selective neurons were distributed equally between chocolate (choc. )- and vanilla (van. )-preferring, and between big- and small-preferring. Shown are flavour- and number-selectivity indices calculated for each recorded neuron, colour-coded as in b . The proportions of significant neurons were not significantly different between small versus big or between choc. versus van. by χ 2 test. Big-preferring, 126 neurons; small-preferring, 152 neurons ( χ 2 stat: 2.4, P =0.12); choc.-preferring, 103 neurons; van.-preferring, 95 neurons ( χ 2 stat: 0.3, P =0.57). Average magnitude of number index for large-preferring versus small-preferring ( t 276 =−1.2, P =0.24); average magnitude of flavour index for choc.-preferring versus van.-preferring ( t 196 =1.1, P =0.29). ( d – f ) Each plot shows, for a single-unit example, average firing rate for each of the four number/flavour combinations, separately for the left and right wells and aligned on initial reward delivery (at 0 s). Vertical dotted lines show epoch from well-entry to reward delivery. ( d ) An example with number/flavour interaction, ( e ) an example with only a number effect and ( f ) an example with only a flavour effect. All examples shown here have strong effects of location. Full size image To determine whether neurons in these anticipatory populations encoded reward value or simply the features of available rewards, we calculated a number and flavour index for each neuron. This index was simply the difference in average peak-normalized firing rate during the reward anticipatory epoch, between the large and small or the chocolate and vanilla reward trials, respectively. As shown in Fig. 2c , both number- and flavour-selective populations were equally distributed between their two poles, indicating that OFC neurons were equally likely to fire selectively in anticipation of large versus small rewards or chocolate versus vanilla rewards (large, 126 neurons; small, 152 neurons; chocolate, 103 neurons; vanilla, 95 neurons). In addition, the average magnitude of the number index did not differ between large- and small-preferring populations, nor did the magnitude of the flavour index differ between chocolate- and vanilla-preferring populations. Thus, OFC seemed to contain similar representations of each variable reward feature, independent of their value relevance as indexed by behaviour. We next asked how these neurons changed their firing rates across number and flavour transitions. Because we were particularly interested in whether they would signal information about expected outcomes before direct experience with them in a new block, we took advantage of one salient feature of our task, which was that a change in reward on one side could be used to predict the features of the new reward on the other side. For example, the sudden receipt of a large chocolate reward on the left meant that a small vanilla reward would now be available on the right. Thus, when a rat received a new reward on one side at the beginning of a new block, it could immediately infer the features—both size and flavour—of the new reward available on the other side. To test whether this inference was evident in the firing rate of outcome-anticipatory OFC neurons, we identified which direction the rats had first received reward after each block switch, and then examined neural activity on the first response in the other direction—that is, the first trial in the off-direction. For simplicity, we will call this trial the ‘inference trial’. We eliminated all cases in which a free-choice trial occurred before the inference trial on the same side, because that free-choice trial would have had the same reward as one on the inference trial. Across all block switches, an average of 2.1±0.1 rewarded trials occurred in the first direction before the critical inference trial occurred in the off-direction. We examined activity in all neurons that were number- or flavour-anticipatory by an ANOVA, using only trials in the second half of blocks (so as not to pre-select the population for early-block selectivity, which we were examining here). We tested activity across block switches in which a preferred reward feature for a particular neuron occurred in the block before or after the switch, comparing the firing rate on the inference trial with that at the end of the previous block (see Methods). If the population signalled the inference, then in the latter case (preferred feature after switch) firing rate might be expected to increase on the inference trial, whereas in the former case (preferred feature before switch) firing rate might be expected to decrease on the inference trial. As illustrated in Fig. 3 for single-unit examples and Fig. 4 for the population, we found exactly this pattern of firing for both number- and flavour-selective neurons. For example, the unit in 3A was selective late in blocks for the small reward (1 drop) at the left well. When the reward on the left changed from three drops to one drop, the neuron fired phasically in anticipation of the new small reward the first time one drop was delivered on the left (that is, before it was directly experienced). The only basis for making this prediction would be knowledge of the associative structure of the task in combination with the memory of having received a new three-drop reward at the right well on the past few trials. These two pieces of information could be used by the rat to infer that it would receive a one-drop reward the next time it responded at the left well. Importantly, such changes in firing were only observed on the inference trial; if we instead analysed activity on the final trial of the previous block (that is, one trial before the inference trial), there was no significant change in activity ( Fig. 5 ). Finally, we performed a second control analysis, shown in Fig. 6 , in which number-selective neurons were tested across flavour block switches, and vice versa; neither of these conditions showed an effect of block switch. A direct comparison of the two control conditions with the inference condition also showed that the observed pattern of changes in activity was specific to the inference trial (stats for this comparison are in the legend for Fig. 6 ). 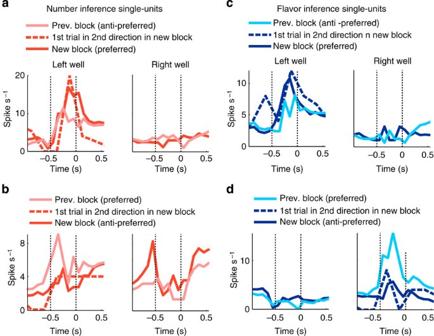Figure 3: Single-unit examples showing inference signalling. (a,b) Number-selective neurons across number block switches and (c,d) flavour-selective neurons across flavour block switches. Plots show average firing rate for the previous (prev.) block (light-coloured line), the new block (dark-coloured line) and the first trial of the new block in the direction that occurred second (the ‘inference trial’; dotted line). Plots are aligned on initial reward delivery (at 0 s); vertical dotted lines show epoch from well-entry to reward delivery. Activity on the opposite side to the inference, in which rewards are always opposite in flavour and number, is also shown. When the block and direction switched from the anti-preferred to preferred reward feature, as in examplesaandc, anticipatory firing on the inference trial tended to be greater than in the prev. block; when it switched from preferred to anti-preferred, as in examplesbandd, anticipatory firing rate on the inference trial tended to be less than in the prev. block. Figure 3: Single-unit examples showing inference signalling. ( a , b ) Number-selective neurons across number block switches and ( c , d ) flavour-selective neurons across flavour block switches. Plots show average firing rate for the previous (prev.) block (light-coloured line), the new block (dark-coloured line) and the first trial of the new block in the direction that occurred second (the ‘inference trial’; dotted line). Plots are aligned on initial reward delivery (at 0 s); vertical dotted lines show epoch from well-entry to reward delivery. Activity on the opposite side to the inference, in which rewards are always opposite in flavour and number, is also shown. When the block and direction switched from the anti-preferred to preferred reward feature, as in examples a and c , anticipatory firing on the inference trial tended to be greater than in the prev. block; when it switched from preferred to anti-preferred, as in examples b and d , anticipatory firing rate on the inference trial tended to be less than in the prev. block. 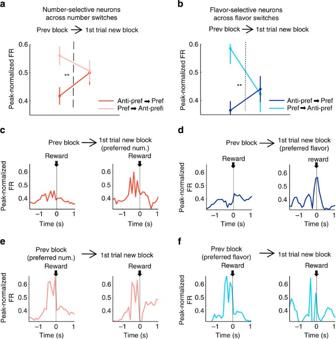Figure 4: Population inference signalling. (a,c,e) Number (num.) switches and (b,d,f) flavour switches. (a,b) Shown is average peak-normalized activity in the 500 ms before reward delivery, for all num.-selective neurons (a) or flavour-selective neurons (b) on the inference trial, compared with the end of the previous block in the same direction. Neurons were separated by whether the new block (dark colour) or previous block (light colour) contained their preferred reward feature. Block switches were only included when the rat had received the new reward at least onceon the opposite sidebefore the first trial shown in this figure. This information would in theory allow the rat to know that a block switch had taken place, and, based on the rules about how rewards were paired in blocks, infer the new reward feature to be presented on that side. The significant interaction between the two conditions (dark- and light-coloured lines) in both num.- and flavour-anticipatory populations indicates that these populations signalled this inference. **Significant interaction atP<0.001 across both populations; see below for detailed statistics. (c–f) Each figure shows population activity across the trial in the conditions summarized inaandb. Incandd, the new block contains the preferred reward feature (dark-coloured line inaandb); phasic activity increased for the new block. Ineandf, the previous block contained the preferred reward feature (light-coloured line inaandb); phasic activity decreased in the new block, especially immediately before reward delivery. Activity in all panels is aligned to the first drop of reward delivery, shown by arrows and dashed lines. ANOVA on anticipatory firing rate across neurons, within-subjects factor before/after, between-subjects factors num./flavour and switch type (anti-preferred→preferred or preferred→anti-preferred): significant interaction between before/after × switch type (F1,320=15.2,P<0.001), with no interaction of this effect with num./flavour (F1,320=1.1,P=0.29). Before/after × switch type interaction was significant for the num.-selective population (F1,320=5.1,P<0.05) and the flavour-selective population (F1,320=10.2,P<0.01). Anti-preferred→preferred increased significantly (F1,320=5.6,P<0.05), with no interaction with num./flavour (F1,320=0.0,P=0.92). Preferred→anti-preferred decreased significantly (F1,320=9.8,P<0.01) with no interaction with num./flavour (F1,320=2.4,P=0.12). Full size image Figure 4: Population inference signalling. ( a , c , e ) Number (num.) switches and ( b , d , f ) flavour switches. ( a , b ) Shown is average peak-normalized activity in the 500 ms before reward delivery, for all num.-selective neurons ( a ) or flavour-selective neurons ( b ) on the inference trial, compared with the end of the previous block in the same direction. Neurons were separated by whether the new block (dark colour) or previous block (light colour) contained their preferred reward feature. Block switches were only included when the rat had received the new reward at least once on the opposite side before the first trial shown in this figure. This information would in theory allow the rat to know that a block switch had taken place, and, based on the rules about how rewards were paired in blocks, infer the new reward feature to be presented on that side. The significant interaction between the two conditions (dark- and light-coloured lines) in both num.- and flavour-anticipatory populations indicates that these populations signalled this inference. **Significant interaction at P <0.001 across both populations; see below for detailed statistics. ( c – f ) Each figure shows population activity across the trial in the conditions summarized in a and b . In c and d , the new block contains the preferred reward feature (dark-coloured line in a and b ); phasic activity increased for the new block. In e and f , the previous block contained the preferred reward feature (light-coloured line in a and b ); phasic activity decreased in the new block, especially immediately before reward delivery. Activity in all panels is aligned to the first drop of reward delivery, shown by arrows and dashed lines. ANOVA on anticipatory firing rate across neurons, within-subjects factor before/after, between-subjects factors num./flavour and switch type (anti-preferred→preferred or preferred→anti-preferred): significant interaction between before/after × switch type (F 1,320 =15.2, P <0.001), with no interaction of this effect with num./flavour (F 1,320 =1.1, P =0.29). Before/after × switch type interaction was significant for the num.-selective population (F 1,320 =5.1, P <0.05) and the flavour-selective population (F 1,320 =10.2, P <0.01). Anti-preferred→preferred increased significantly (F 1,320 =5.6, P <0.05), with no interaction with num./flavour (F 1,320 =0.0, P =0.92). Preferred→anti-preferred decreased significantly (F 1,320 =9.8, P <0.01) with no interaction with num./flavour (F 1,320 =2.4, P =0.12). 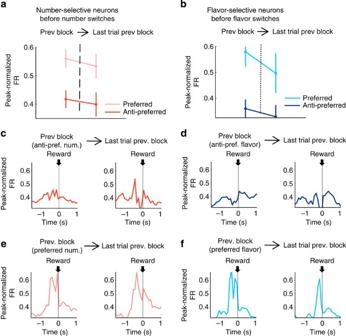Figure 5: Control analysis demonstrating that activity does not change on the last trial before the block switch in the same populations. (a,b) Shown is average peak-normalized activity in the 500 ms before reward delivery, for all number (num.)-selective neurons (a) or flavour-selective neurons (b) on the last trial before the block switch compared with end of that block not including the last trial. This analysis includes the same populations in the same blocks as in the inference analysis, with neurons categorized as anti-preferred (anti-pref.) or preferred in the same way. (c–f) Each panel shows population activity across the trial in the conditions summarized inaandb. Activity in all panels is aligned to reward delivery, shown by arrows and dashed lines. ANOVA on anticipatory firing rate across neurons, with within-subjects factor before/after, and between-subjects factors num./flavour and preferred/anti-preferred. No interaction of before/after × preferred/anti-preferred (F1,320=0.3,P=0.57), and no other effects (Fs<2.3,Ps>0.13). Neither the num.-selective population (F1,320=0.0,P=0.90) nor the flavour-selective population (F1,320=0.4,P=0.53) showed an interaction between before/after × preferred/anti-preferred. At neither the level of preferred nor anti-preferred there was a significant effect of before versus after (F1,320=2.1,P=0.15; F1,320=0.5,P=0.49). Prev, previous. Full size image Figure 5: Control analysis demonstrating that activity does not change on the last trial before the block switch in the same populations. ( a , b ) Shown is average peak-normalized activity in the 500 ms before reward delivery, for all number (num. )-selective neurons ( a ) or flavour-selective neurons ( b ) on the last trial before the block switch compared with end of that block not including the last trial. This analysis includes the same populations in the same blocks as in the inference analysis, with neurons categorized as anti-preferred (anti-pref.) or preferred in the same way. ( c – f ) Each panel shows population activity across the trial in the conditions summarized in a and b . Activity in all panels is aligned to reward delivery, shown by arrows and dashed lines. ANOVA on anticipatory firing rate across neurons, with within-subjects factor before/after, and between-subjects factors num./flavour and preferred/anti-preferred. No interaction of before/after × preferred/anti-preferred (F 1,320 =0.3, P =0.57), and no other effects (Fs<2.3, P s>0.13). Neither the num.-selective population (F 1,320 =0.0, P =0.90) nor the flavour-selective population (F 1,320 =0.4, P =0.53) showed an interaction between before/after × preferred/anti-preferred. At neither the level of preferred nor anti-preferred there was a significant effect of before versus after (F 1,320 =2.1, P =0.15; F 1,320 =0.5, P =0.49). Prev, previous. 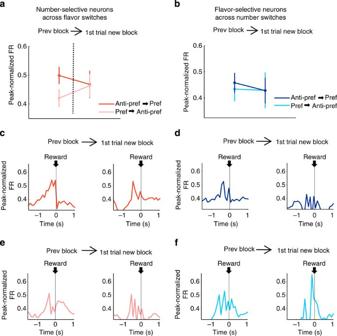Figure 6: Control analysis demonstrating activity across block switches in which the preferred reward feature does not change. (a,b) Shown is average peak-normalized activity of the same populations during the same epoch shown inFig. 4, but here number-anticipatory neurons are shown across flavour switches (a) and flavour-anticipatory neurons across number switches (b). Neurons were separated by whether the inference condition (shown inFig. 4) in the new block and direction contained their preferred reward feature (dark colour) or their anti-preferred reward feature (light colour). Block switches were only included when the rat had received the new reward at least onceon the opposite sidebefore the first trial shown in this figure. (c–f) Each panel shows population activity across the trial in the conditions summarized inaandb. Activity in all panels is aligned to reward delivery, shown by arrows and dashed lines. ANOVA on anticipatory firing rate across neurons, within-subjects factor before/after, and between-subjects factors number/flavour and switch type (anti-preferred→preferred or preferred→anti-preferred): no interaction of before/after × switch type (F1,320=1.0,P=0.32), and no other effects F’s<0.6,P’s>0.45). Neither the number-selective population (F1,320=1.4,P=0.23) nor the flavour-selective population (F1,320=0.1,P=0.74) showed an interaction between before/after × switch type. To compare the two control conditions (Figs 5and6) with the inference condition, we ran an ANOVA on the difference scores (after-before) for the inference condition, first control condition (Fig. 5) and second control condition (Fig. 6), as a within-subjects factor, and switch type (anti-preferred → preferred or preferred → anti-preferred), as a between-subjects factor. This ANOVA revealed an interaction between difference-score and switch-type (F2,644=6.3,P=0.002). The interaction between inference versus the two controls (pooled) × switch-type was also significant (planned comparison: F1,322=12.2,P=0.0006). And, at each level of switch-type, the comparison of inference versus the two controls was also significant (planned comparisons: anti-preferred to preferred, F1,322=8.2,P=0.004; preferred to anti-preferred, F1,322=4.3,P=0.039). Full size image Figure 6: Control analysis demonstrating activity across block switches in which the preferred reward feature does not change. ( a , b ) Shown is average peak-normalized activity of the same populations during the same epoch shown in Fig. 4 , but here number-anticipatory neurons are shown across flavour switches ( a ) and flavour-anticipatory neurons across number switches ( b ). Neurons were separated by whether the inference condition (shown in Fig. 4 ) in the new block and direction contained their preferred reward feature (dark colour) or their anti-preferred reward feature (light colour). Block switches were only included when the rat had received the new reward at least once on the opposite side before the first trial shown in this figure. ( c – f ) Each panel shows population activity across the trial in the conditions summarized in a and b . Activity in all panels is aligned to reward delivery, shown by arrows and dashed lines. ANOVA on anticipatory firing rate across neurons, within-subjects factor before/after, and between-subjects factors number/flavour and switch type (anti-preferred→preferred or preferred→anti-preferred): no interaction of before/after × switch type (F 1,320 =1.0, P =0.32), and no other effects F’s<0.6, P ’s>0.45). Neither the number-selective population (F 1,320 =1.4, P =0.23) nor the flavour-selective population (F 1,320 =0.1, P =0.74) showed an interaction between before/after × switch type. To compare the two control conditions ( Figs 5 and 6 ) with the inference condition, we ran an ANOVA on the difference scores (after-before) for the inference condition, first control condition ( Fig. 5 ) and second control condition ( Fig. 6 ), as a within-subjects factor, and switch type (anti-preferred → preferred or preferred → anti-preferred), as a between-subjects factor. This ANOVA revealed an interaction between difference-score and switch-type (F 2,644 =6.3, P =0.002). The interaction between inference versus the two controls (pooled) × switch-type was also significant (planned comparison: F 1,322 =12.2, P =0.0006). And, at each level of switch-type, the comparison of inference versus the two controls was also significant (planned comparisons: anti-preferred to preferred, F 1,322 =8.2, P =0.004; preferred to anti-preferred, F 1,322 =4.3, P =0.039). Full size image Interestingly, the inference signal observed in OFC neurons was not tightly locked to the rats’ behaviour. For number switches, OFC neurons seemed to infer the outcome before the rats’ behaviour clearly reflected this knowledge, at least according to our standard behavioural metrics. Rats took about 12 rewarded trials (6 in each direction) after a block switch to reach a 50% choice rate (that is, choosing both sides equally). In contrast, the inference signal was detectable before the first time a new reward was delivered in the off-direction. In addition, for flavour switches, the inference signal seemed to be completely dissociated from behaviour, because rats did not change their behaviour in any obvious way in response to flavour changes. This suggests that the neural inference signal was not a consequence of behaviour, but it also calls into question whether the signal has any behavioural relevance. To examine this issue, we looked at choice rate on blocks in which we observed strong inference signals versus those in which we observed weak inference signals, by calculating an inference score for each number-selective neuron across each included block switch. This score was simply the difference between the normalized firing rate on the inference trial of the new block minus that in the same direction at the end of the previous block (see Methods). As shown in Fig. 7a , when the number of drops changed, a large inference score was associated with a rapid switch in choice behaviour. This difference was most pronounced in the first five trials of the block, but was significant until about trial ten. Accordingly, across the first ten trials of the block, we found a significant positive correlation between the neural inference score of the single-units and the rats’ choice rates ( R =0.28, P <0.01, Pearson correlation). This correlation was specific for activity on the inference trial. As shown in Fig. 7b , when we did a parallel analysis using the last trial of the previous block in place of the inference trial, there was no correlation with choice behaviour in the new block ( R =−0.031, P =0.75, Pearson correlation). 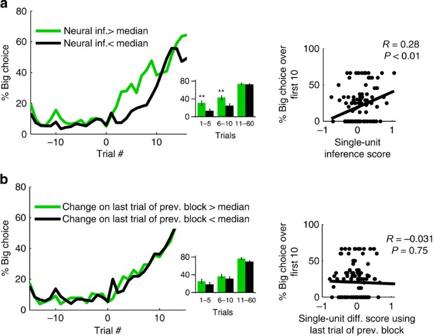Figure 7: Neural inference signals positively correlate with the rate at which choice behaviour adjusts to the block switch. (a) Shown is the average trial-by-trial choice rate across number block switches when a neuron with an inference scoreabove(green line) orbelow (black line) the median was recorded. Inset shows average choice rate across the first 5 trials, next 5 trials or trials 11–60. Scatter plot shows the correlation between the single-unit inference score (difference in normalized firing rate between inference trial and end of previous (prev.) block; see Methods) and choice rate over the first ten trials. Choice rate is defined as the percentage of choices towards the side with the big reward in the new block. ANOVA on choice rate with factors group and trial-set (1–5, 6–10 or 11–60), found a significant effect of group (F1,513=17.6,P<0.0001) and a group × trial-set interaction (F2,513=3.6,P<0.05), planned comparisons between groups were significant at trials 1–5 (F1,513=10.7,P<0.01), trials 6–10 (F1,513=12.3,P<0.001), but not at trials 11–60 (F1,513=0.1,P=0.76). **P<0.01. (b) For this control analysis, activity on the last forced-choice trial before the block switch was used to compute the difference score (difference in normalized firing rate between that trial and trials at the end of that block not including that trial). ANOVA on choice rate with factors group and trial-set (1–5, 6–10 or 11–60), found a small effect of group (F1,513=4.3,P<0.05), but no group × trial-set interaction (F2,513=0.0,P=0.96) and no effect of group at any level of trial-set (F’s<2.1,P’s>0.15) inf, Inference. Figure 7: Neural inference signals positively correlate with the rate at which choice behaviour adjusts to the block switch. ( a ) Shown is the average trial-by-trial choice rate across number block switches when a neuron with an inference score above (green line) or below ( black line) the median was recorded. Inset shows average choice rate across the first 5 trials, next 5 trials or trials 11–60. Scatter plot shows the correlation between the single-unit inference score (difference in normalized firing rate between inference trial and end of previous (prev.) block; see Methods) and choice rate over the first ten trials. Choice rate is defined as the percentage of choices towards the side with the big reward in the new block. ANOVA on choice rate with factors group and trial-set (1–5, 6–10 or 11–60), found a significant effect of group (F 1,513 =17.6, P <0.0001) and a group × trial-set interaction (F 2,513 =3.6, P <0.05), planned comparisons between groups were significant at trials 1–5 (F 1,513 =10.7, P <0.01), trials 6–10 (F 1,513 =12.3, P <0.001), but not at trials 11–60 (F 1,513 =0.1, P =0.76). ** P <0.01. ( b ) For this control analysis, activity on the last forced-choice trial before the block switch was used to compute the difference score (difference in normalized firing rate between that trial and trials at the end of that block not including that trial). ANOVA on choice rate with factors group and trial-set (1–5, 6–10 or 11–60), found a small effect of group (F 1,513 =4.3, P <0.05), but no group × trial-set interaction (F 2,513 =0.0, P =0.96) and no effect of group at any level of trial-set (F’s<2.1, P ’s>0.15) inf, Inference. Full size image The relationship between the inference signal and the rats’ choice performance can also be shown if we divide sessions by whether the rats switched quickly to the large reward at the start of the block (choice rate in first ten trials above the median) or only more slowly (choice rate in first ten trials below the median). As illustrated in Fig. 8 , this analysis shows that neural inference was only observed at the start of fast-switching blocks and not at all at the start of slow-switching blocks. Again, this difference was specific for the inference trial: when we compared activity either on the last trial of the previous block or at the end of the new block, fast-switching and slow-switching blocks did not differ in OFC reward selectivity. 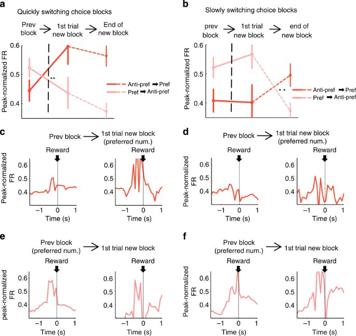Figure 8: OFC number-selective neurons signal the inference only on blocks in which the rat subsequently switches choice behaviour quickly. (a,b) Shown is average peak-normalized activity of all number (num.)-anticipatory neurons, as inFig. 4, here separated by whether choice rate on the first ten trials wasabove(a) orbelow(b) the median. Dotted line shows activity at the end of the block in the same direction. The two groups differed in selectivity on the inference trial, but not on the trial immediately before it (the last trial in the previous (prev.) block, not shown here) nor at the end of the block. **Significant interaction atP<0.01 (see below for detailed statistics). (c–f) Each panel shows population activity across the trial in the conditions summarized inaandb. Activity in all panels is aligned to reward delivery, shown by arrows and dashed lines. ANOVA on difference in firing rate from the end of the prev. block, factors: trial (last trial of prev. block, inference trial, end of new block), switch type (anti-preferred (anti-pref.)→preferred/preferred→anti-pref.) and group (fast-switching/slow-switching), found a significant three-way interaction (F2,366=3.9,P<0.05). In the fast-switching group, effect of switch type was significant on last trial (F1,183=0.3,P=0.60), but not on inference trial (F1,183=10.7,P<0.01) nor at end (F1,183=58.5,P<0.0001). For the slow-switching group, no effect of switch type on last trial (F1,183=0.2,P=0.67) nor inference trial (F1,183=0.5,P=0.48) but a significant effect at end (F1,183=44.0,P<0.0001). Interaction between group × switch type was not significant on last trial (F1,183=0.0,P=0.94) nor at end (F1,183=0.4,P=0.52), but was on inference trial (F1,183=7.9,P<0.01). Inference trial versus end of the new block × switch type interaction was not significant for the fast-switching group (F1,183=0.2,P=0.65), but was significant for the slow-switching group (F1,183=17.4,P<0.0001); interaction between these interactions was significant (F1,183=7.0,P<0.01). No effect of group and no group × preferred versus anti-pref. interaction on firing rate at the end of the prev. block (leftmost points in top panels; F1,183=0.3,P=0.60; F1,183=0.2,P=0.63) FR, firing rate. Figure 8: OFC number-selective neurons signal the inference only on blocks in which the rat subsequently switches choice behaviour quickly. ( a , b ) Shown is average peak-normalized activity of all number (num. )-anticipatory neurons, as in Fig. 4 , here separated by whether choice rate on the first ten trials was above ( a ) or below ( b ) the median. Dotted line shows activity at the end of the block in the same direction. The two groups differed in selectivity on the inference trial, but not on the trial immediately before it (the last trial in the previous (prev.) block, not shown here) nor at the end of the block. **Significant interaction at P <0.01 (see below for detailed statistics). ( c – f ) Each panel shows population activity across the trial in the conditions summarized in a and b . Activity in all panels is aligned to reward delivery, shown by arrows and dashed lines. ANOVA on difference in firing rate from the end of the prev. block, factors: trial (last trial of prev. block, inference trial, end of new block), switch type (anti-preferred (anti-pref.)→preferred/preferred→anti-pref.) and group (fast-switching/slow-switching), found a significant three-way interaction (F 2,366 =3.9, P <0.05). In the fast-switching group, effect of switch type was significant on last trial (F 1,183 =0.3, P =0.60), but not on inference trial (F 1,183 =10.7, P <0.01) nor at end (F 1,183 =58.5, P <0.0001). For the slow-switching group, no effect of switch type on last trial (F 1,183 =0.2, P =0.67) nor inference trial (F 1,183 =0.5, P =0.48) but a significant effect at end (F 1,183 =44.0, P <0.0001). Interaction between group × switch type was not significant on last trial (F 1,183 =0.0, P =0.94) nor at end (F 1,183 =0.4, P =0.52), but was on inference trial (F 1,183 =7.9, P <0.01). Inference trial versus end of the new block × switch type interaction was not significant for the fast-switching group (F 1,183 =0.2, P =0.65), but was significant for the slow-switching group (F 1,183 =17.4, P <0.0001); interaction between these interactions was significant (F 1,183 =7.0, P <0.01). No effect of group and no group × preferred versus anti-pref. interaction on firing rate at the end of the prev. block (leftmost points in top panels; F 1,183 =0.3, P =0.60; F 1,183 =0.2, P =0.63) FR, firing rate. Full size image Given the relationship between the number inference signal and behaviour, we next wondered whether flavour inferences had any relationship with behaviour. Although flavour changes had no enduring effect on choice rate, a small downward deflection in choice rate appeared to occur immediately after flavour switches ( Fig. 1c ). We tested whether this change was significant by examining choice rate in the first two free-choice trials after flavour switches. Indeed, there was a small but significant decrease in the choice rate towards the large reward (or, equivalently, an increase in choice rate towards small reward) in those first two free-choice trials, as compared with the last two free-choice trials of the previous block. This difference disappeared in the next two free-choice trials of the new block (last two choice trials of previous block: 15±2.0% small choice; first two of new block: 22±2.5%; next two of new block: 17±2.3%; a within-subjects ANOVA on choice rate, with factor trial-pair found a main effect of trial pair: F 2,374 =3.2, P <0.05; planned comparison between last two trials and first two trials: F 1,187 =6.3, P <0.05; planned comparison between last two trials and second two trials: F 1,187 =0.5, P =0.47). To test whether this behavioural effect of flavour switches was related to the flavour inference neural signal, we divided flavour block switches by whether the first two free-choice trials after the switch had at least one choice of the small reward, or whether they had none (this split was in effect a median split, because the median number of small choices in the first two was zero). We re-examined neural activity in the same flavour anticipatory population analysed earlier across flavour switches, this time testing each side of the split separately. As shown in Fig. 9 , in the small-choice group, inference signalling was significant on the inference trial, but did not change significantly between the inference trial and the end of the block. Conversely, in the zero-small-choice group, neurons did not show significant changes in activity on the inference trial, and all updating occurred between the inference trial and the end of the new block. Thus, like number inference signalling, strong flavour inference signalling appears to be associated with a behavioural change that may indicate immediate awareness of the switch. However, we did not see a significant interaction between group and signalling on the inference trial, indicating that this behavioural measure was not as closely tied to behaviour as the speed of choice updating was. We were also unable to test for a correlation with this behaviour, because almost all switches had either zero small choices or one small choice within these two free-choice trials. 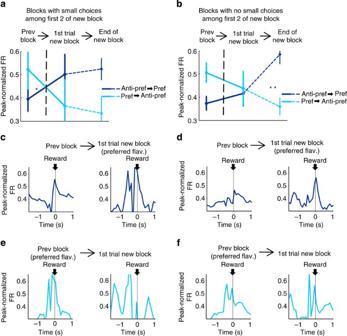Figure 9: OFC flavour (flav)-selective neurons signal the inference only on blocks in which the rat chooses the small reward. (a,b) Shown is average peak-normalized activity of all flav.-anticipatory neurons, as inFig. 4, here separated by whether rats chose small reward on one of the first two free-choice trials of the new block (a) or on neither (b). Dotted line shows activity at the end of the block in the same direction. Choosing small reward may indicate immediate awareness of the block switch (see Results). Ina, all significant updating occurred on the inference trial, whereas inb, all significant updating occurred between the inference trial and the end of the block. *,**Significant interaction atP<0.05 orP<0.01, respectively (see below for detailed statistics). (c–f) Each panel shows population activity across the trial in the conditions summarized inaandb. Activity in all panels is aligned to reward delivery, shown by arrows and dashed lines. ANOVA on difference in firing rate from the end of the previous (prev.) block, with factors trial (last trial of prev. block, inference trial, end of new block), switch type (anti-preferred→preferred or preferred→anti-preferred) and group (small-choice/no-small-choice), found a trend towards a significant effect of group (F1,126=3.3,P=0.071). In the small-choice group, effect of switch type was not significant on last trial (F1,126=2.0,P=0.16), but was significant on inference trial (F1,126=4.0,P<0.05) and at end (F1,126=19.9,P<0.0001). For the no small-choice group, effect of switch type not significant on last trial (F1,126=0.3,P=0.62) nor inference trial (F1,126=2.1,P=0.15) but was at end (F1,126=76.5,P<0.00001). No significant group × switch type interactions at any level of trial (F’s<2.2,P’s>0.13). Inference trial versus end × switch type interaction was not significant for the small-choice group (F1,126=0.1,P=0.71), but was significant for the no-small-choice group (F1,126=9.1,P<0.003); interaction between these interactions was not significant (F1,126=1.4,P=0.24). No effect of group on firing rate at the end of the prev. block (leftmost points in top panels; F1,126=0.1,P=0.71) and no group × preferred versus anti-preferred interaction at the end of the prev. block (F1,183=0.0,P=0.97). Figure 9: OFC flavour (flav)-selective neurons signal the inference only on blocks in which the rat chooses the small reward. ( a , b ) Shown is average peak-normalized activity of all flav.-anticipatory neurons, as in Fig. 4 , here separated by whether rats chose small reward on one of the first two free-choice trials of the new block ( a ) or on neither ( b ). Dotted line shows activity at the end of the block in the same direction. Choosing small reward may indicate immediate awareness of the block switch (see Results). In a , all significant updating occurred on the inference trial, whereas in b , all significant updating occurred between the inference trial and the end of the block. *,**Significant interaction at P <0.05 or P <0.01, respectively (see below for detailed statistics). ( c – f ) Each panel shows population activity across the trial in the conditions summarized in a and b . Activity in all panels is aligned to reward delivery, shown by arrows and dashed lines. ANOVA on difference in firing rate from the end of the previous (prev.) block, with factors trial (last trial of prev. block, inference trial, end of new block), switch type (anti-preferred→preferred or preferred→anti-preferred) and group (small-choice/no-small-choice), found a trend towards a significant effect of group (F 1,126 =3.3, P =0.071). In the small-choice group, effect of switch type was not significant on last trial (F 1,126 =2.0, P =0.16), but was significant on inference trial (F 1,126 =4.0, P <0.05) and at end (F 1,126 =19.9, P <0.0001). For the no small-choice group, effect of switch type not significant on last trial (F 1,126 =0.3, P =0.62) nor inference trial (F 1,126 =2.1, P =0.15) but was at end (F 1,126 =76.5, P <0.00001). No significant group × switch type interactions at any level of trial (F’s<2.2, P ’s>0.13). Inference trial versus end × switch type interaction was not significant for the small-choice group (F 1,126 =0.1, P =0.71), but was significant for the no-small-choice group (F 1,126 =9.1, P <0.003); interaction between these interactions was not significant (F 1,126 =1.4, P =0.24). No effect of group on firing rate at the end of the prev. block (leftmost points in top panels; F 1,126 =0.1, P =0.71) and no group × preferred versus anti-preferred interaction at the end of the prev. block (F 1,183 =0.0, P =0.97). Full size image The question of whether inference signalling reflects partial or complete updating of the number or flavour selectivity can be answered using the split data described above. For both number and flavour block switches, when rats showed behavioural evidence of being aware of the block change (that is, either fast choice switching after number switches or transient small-choices after flavour switches), no significant additional updating occurred between the inference trial and the end of the new block. Conversely, when there was less evidence that rats were aware of the block change, the inference trial itself showed no evidence of updating, and instead all significant updating happened between the inference trial and the end of the new block. Finally, we asked whether any behavioural or neural factor might predict the strength of either the drop-number or flavour inference signal. We examined (i) the total number of trials in the previous block, (ii) the percent of block switches that were the first switch of the session, (iii) the choice rate at the end of the previous block and (iv) the total number of errors in the previous block. As detailed in Table 1 , none of these factors were significantly different between block switches in which the inference signal was above the median as compared with when it was below the median. Likewise, as illustrated in the leftmost points in the top panels of Figs 8 and 9 , the strength of drop-number or flavour selectivity at the end of the previous block failed to predict whether rats would switch choice rate quickly in the new block (for drop-number switches), or whether the first two free-choice trials would contain a small choice (for flavour switches). Table 1 Behavioural variables from the block previous to block switches in which inference signals are greater or less than the median. Full size table The ability to predict likely outcomes or consequences is fundamental to normal adaptive behaviour and learning. This ability obviously benefits if changes in outcomes can be inferred based on an understanding of the rules or causal structure of the environment rather than requiring direct experience. Broadly speaking, this is the basis of the distinction between so-called habitual or model-free behaviour, in which responses are made based on pre-computed or cached values or ‘policies’, and goal-directed, outcome-guided or model-based behaviour, in which responses are based on values or policies that are arrived at on-the-fly through a process of mental simulation [24] , [25] , [26] , [27] . Historically, the OFC has been strongly associated with emotions and associative behaviour [28] , [29] , [30] ; however, in the past decade, accounts of this involvement have been increasingly dichotomized to reflect the division between signalling information derived solely from direct experience versus information that is inferred from access to relationships between events in the environment or task at hand. OFC is typically not necessary for the former but is always critical for the latter [13] , [18] , [20] , [21] , [22] , [23] . This has been interpreted as showing a role for the OFC in signalling an inferred or derived rather than a pre-computed value [6] , [13] . Yet a growing number of accounts implicate the OFC not only in signalling inferred value but also in signalling value-independent information about impending events. This is evident in single unit and functional magnetic resonance imaging studies, in which neural signals in OFC represent features of impending outcomes—and in fact other predictable events—even when they are value neutral [6] , [11] , [14] , [15] , [31] . And in rats there exists clear evidence that the OFC is necessary for behaviour and learning that reflects these specific sensory features [18] , [19] , [32] . These data raise the possibility that the OFC may not only represent value, even inferred, but also instead may be a fundamental part of the circuit that represents the associative structure of the environment [33] . Here we provide single-unit evidence consistent with this proposal. Specifically, we found that single units in rat OFC fired in anticipation of expected outcomes in a way that reflected both value-based and value-neutral features of the outcomes. Indeed, the strength or directionality of the correlates did not appear to be especially tied to whether or not the features had implications for value. As such, these results are consistent with a variety of prior reports that have emphasized the signalling of value-neutral associative features in the OFC [11] , [15] , [16] , [17] . Of course, information about value-neutral features could still be used to derive value or to drive goal-directed behaviour, but regardless of its use, these results suggest that OFC neurons represent a rich description of the specific features defining the outcome, including even the location or directional response required to obtain it. Furthermore, this information was represented immediately at the start of new trial blocks, even before the predicted outcome features had been directly re-experienced. As noted earlier, such a prediction would require knowledge of the rules or associative structure of the task. Rats may use this knowledge to mentally simulate predicted outcomes (as model-based processing is usually conceived) or, alternatively, they may recognize which of the unique task ‘states’ (that is, the arrangement of outcomes in each block) they are currently in. Notably, both approaches require rats to represent the ‘state space’ or, equivalently, the associative structure of the task, in concert with more local information (recently experienced outcomes), to make predictions that in turn allow fast updating of choice behaviour. This linking together of associative information to promote flexible responding is consistent with the proposal that the OFC is part of a network involved in tracking hidden environmental states and making predictions about impending events [33] . This role may be one reason the OFC is important for behaviour in settings similar to the current task, which involve reversals [21] , [30] , [34] , [35] , [36] , however, it may also be related to OFC’s involvement in flexible behaviour that goes beyond immediate or even direct experience [37] , [38] , [39] , [40] , [41] . Subjects Male Long-Evans rats were obtained at 175–200 g (~60 days old on arrival) from Charles River Labs. Rats were tested at the University of Maryland School of Medicine in accordance with School of Medicine and NIH guidelines. Surgical procedures and histology Surgical procedures followed guidelines for aseptic technique. Electrodes, consisting of drivable bundles of eight 25-μm diameter FeNiCr wires (Stablohm 675, California Fine Wire) electroplated with platinum to an impedance of ~300 kΩ, were manufactured and implanted as in prior recording experiments. Driveable electrodes were implanted in the left OFC ( n =6; 3.0 mm anterior to bregma, 3.2 mm laterally, and, to begin, 4.0 mm ventral to the surface of the brain) in each rat. Four rats also had electrodes implanted in the ventral striatum; those data are not included in this report. At the end of the study, the final electrode position was marked, the rats were euthanized with an overdose of isoflurane and perfused, and the brains were removed from the skulls and processed using standard techniques. Behavioural task Recording was conducted in aluminium chambers, on one wall of which was a panel with an odour port and two fluid wells arranged below it (see Fig. 1 ). The odour port was connected to an air flow dilution olfactometer to allow the rapid delivery of olfactory cues. The fluid wells were connected to fluid delivery lines containing flavoured milk (Nesquick brand chocolate or vanilla) diluted 50% with water. Delivery of odours at the odour port and the fluids at the fluid wells was controlled by a custom C++ programme interfaced with solenoid valves. Photobeam breaks at the port and wells were monitored and recorded by the programme. A houselight was also controlled by the programme. Rats were trained extensively before implanting them with electrodes. After implantation, we retrained rats to work with the recording cable. Each training session included as many trials as a rat would perform before quitting, approximately 150–250. This initial shaping phase gradually introduced all elements of the task (described below), and thus rats could learn the associative structure of the task over this period. Recording was begun when rats could complete five blocks of trials (at least 260 trials) with the cable. Total number of pre-recording training sessions averaged 32.5 (ranging from 24 to 43). Each recording session consisted of a series of self-paced trials organized into five blocks. Rats could initiate a trial by poking into the odour port while the house light was illuminated. Beginning 500 ms after the odour poke, an odour would be delivered for 500 ms. If the rat withdrew from the odour port before completion of the 1,000 ms pre-odour+odour period, the trial would be aborted and the houselight turned off. At the end of the odour, rats could respond by moving from the odour port to the left fluid well or the right fluid well, after which they had to wait for 500 ms before fluid delivery began; if they exited the well during this period, no fluid was delivered and the trial ended. The identity of the odour specified whether they could receive reward at the left well (forced-choice left), the right well (forced-choice right) or either well (free-choice). The identity and meaning of these odours remained the same across the entire experiment. Odours were presented in a pseudorandom sequence such that the free-choice odour was presented on 7/20 trials and the left/right odours were presented in equal numbers (±1 over 250 trials). In addition, the same odour could be presented on no more than three consecutive trials. Rewards were either one bolus or three boli of chocolate or vanilla milk, with bolus size ~0.05 ml and 500 ms between boli. Response-reward contingencies were consistent within blocks of trials, such that the same reward would be delivered for every correct right response, either free or forced choice, and a different reward would be delivered for every correct left response, free or forced choice. The reward schedule was arranged so that in each block, reward features available on one side were always paired with the opposite reward features on the other side—thus when one drop of chocolate milk was available on the left, three drops of vanilla was available on the right, and so on, resulting in a total of four different reward combinations. On the first block, consisting of on average 43 (standard deviation 16) trials that were used to set the rats’ expectations before the first block switch, one of these combinations was randomly chosen. The subsequent four block transitions then followed, in order: (i) a drop-number transition, in which the side with one drop changed to three drops and vice versa, but the side-flavour contingencies remained the same; (ii) a flavour transition, in which the side with chocolate changed to vanilla and vice versa, but the side-number contingencies remained the same, (iii) another drop-number transition, (iv) another flavour transition. These block transitions were not explicitly signalled. The length of the last four blocks varied non-systematically around 65, with a standard deviation of 10.7 across the experiment. During testing, rats were limited to 10 min of ad lib water each day, in addition to fluid earned in the task. Flavour preference testing In six rats from a separate experiment (same strain and source, and same water restriction regimen), we compared consumption of the chocolate versus vanilla milk solution in two-bottle tests. All rats were tested for total 10 min, with the location of the bottles swapped every 30 s. Two rats were given five 2-min tests, whereas the other four rats were given one 10-min test each. Single-unit recording Procedures were the same as described previously [42] . Wires were screened for activity daily; if no activity was detected, the rat was removed and the electrode assembly was advanced 40 or 80 μm. Otherwise a session was conducted, and the electrode was advanced by at least 40 μm at the end of the session. Neural activity was recorded using Plexon Multichannel Acquisition Processor systems (Plexon Inc.), interfaced with odour discrimination training chambers. Signals from the electrode wires were amplified and filtered by standard procedures described in the previous studies. Waveforms (>2.5:1 signal-to-noise) were extracted from active channels and recorded with event timestamps sent by the behavioural programme. Waveforms were not inverted before data analysis. Data analysis Units were sorted using Offline Sorter software from Plexon Inc., using a template-matching algorithm. Sorted files were then processed in Neuroexplorer to extract unit timestamps and relevant event markers. These data were subsequently analysed in Matlab. To analyse reward anticipatory activity, we examined firing rate in the 500 ms epoch between fluid well entry and the first bolus of reward delivery. We performed an ANOVA ( P <0.05) on each neuron’s firing rate during this epoch, with baseline (from houselight on to odour initiation) subtracted, using factors number of reward drops (one or three), reward flavour (chocolate or vanilla) and well location (left or right). In the initial ANOVA, we included all correct forced-choice trials across the last four blocks (across which all factors were completely crossed and balanced). Every neuron with a number or flavour effect, regardless of whether it showed an inhibitory or excitatory response, was included. To measure the degree of number- and flavour-selectivity, we calculated a number and flavour index for each neuron. To do so, we peak-normalized each neuron by dividing all firing rates by a normalization factor, which was the peak firing rate across the trial in 500 ms bins after averaging across the first ten and last ten of each of the eight number-flavour-well conditions in the last four blocks. We then calculated the number and flavour indices as: 1 number index=average peak-normalized firing rate on all three-drop trials−average peak-normalized firing rate on all one-drop trials 2 flavour index=average peak-normalized firing rate on all chocolate trials−average peak-normalized firing rate on all vanilla trials. For neurons with significant interaction effects, the above formulas would not reflect the actual degree of their selectivity, so for those neurons, we calculated separate indices for each level of the interacting factor, and then took the index with the highest absolute value. For instance, for a neuron with a flavour × direction interaction, we calculated separate flavour indices for the left and right wells, and then assigned whichever of these was greater in magnitude as the flavour index for that neuron. To analyse neural activity reflecting inferences, we identified the well at which reward was first delivered after each block switch, and then identified the first forced-choice trial that was rewarded at the other well in that block, eliminating cases in which a free-choice trial was rewarded at that well before the first forced-choice trial. For simplicity, we will call this trial the inference trial. The inference trial was therefore the first trial of the block in which reward was delivered at that well. We compared reward-anticipatory activity on the inference trial with activity in forced-choice trials in the same direction at the end of the previous block. For the reported analysis, this previous block activity was the average of the last three trials, not including the last one, from the previous block, but the results remained qualitatively the same independent of exactly how many trials from the previous block we used; we eliminated the last trial so that we could examine activity on that trial as a control. For drop-number-selective neurons, we noticed that they tended to ramp up firing before the rat entered the fluid well to wait for reward; thus we changed the epoch to begin 100 ms before fluid well entry, still ending upon delivery of the first drop of reward. To define the population to be tested for inference signalling, we first redid the ANOVA, this time only including forced-choice trials after the first 20 in each block (the last half of blocks). We did this in order to eliminate statistical bias towards finding inference, which would occur at the beginning of blocks, but results were similar using the original ANOVA. We tested for inference signalling across all neurons with a significant effect of number, flavour or interactions of these factors. Each neuron’s preferred reward feature was defined for main effect neurons as the feature it fired most for across the trials that went into the ANOVA. For instance, for a neuron with a main effect of number, it was defined as three-drop preferring if it fired most across trials (after the first 20 of blocks) in which the three-drop reward was delivered. For interaction effects, we did follow-up ANOVAs at each level of the interacting factor to determine whether that neuron had a significant effect at each level, and, if so, which reward feature it preferred at that level. For instance, for a neuron with a significant flavour × direction effect, we tested for a flavour effect separately at the left well and the right well, and, for each significant effect, defined whether that neuron preferred chocolate or vanilla at that well. Then, for inference testing, we only included a neuron when the block transition in the analysed direction consisted of a switch between that neurons preferred to anti-preferred reward feature, or between its anti-preferred to preferred reward feature. We also did two control analyses to test whether observed patterns of changes were specific to inference: (i) for each neuron, we replaced the inference trial with final trial of the previous block, but leaving all other factors the same, and (ii) for each neuron, we examined the change across the opposite block change from that in which the inferential change was measured (for example, for a flavour inference measured on the first flavour block change, we examined its change across the first number block change). For correlations with behaviour, we calculated an inference score for each neuron across each qualifying block switch, defined as follows: 1 inference score=(sign-factor)*(peak-normalized firing rate during the analysed epoch of the inference trial−average peak-normalized firing rate in the analysed epoch over the last 10 (not including the last trial) of the previous block in the same direction.) 2 sign-factor=1, for anti-preferred → preferred switches 3 sign-factor=−1, for preferred → anti-preferred switches We used ten trials from the previous block in equation 3 in order to reduce trial-to-trial variability in the score as much as possible, but, again, the exact number of trials from the previous block did not change the results qualitatively. As a control, we tested a parallel correlation in which we substituted for the inference trial the last forced-choice trial from the previous block. We also calculated selectivity at the end of the new block, in parallel to the inference score, as follows: 1 end-of-block selectivity=(sign-factor)*(average peak-normalized firing rate in the last 10 (not including the last trial) of the new block in the same direction as the inference trial−average peak-normalized firing rate over the last 10 (not including the last trial) of the previous block in the same direction). When data for correlations contained two block changes for the same neuron, those data points were averaged so that each data point in the correlation came from a unique neuron. Statistics were done using Matlab, Excel and Statistica. Planned comparisons were used for testing specific effects of multi-way ANOVAs. For displays of neural activity, bin-size was 100 ms except when the inference trial was shown for single-units, in which case bin-size was 250 ms. Neural activity in the displays was smoothed with a boxcar algorithm, with a 9-bin boxcar used for single-unit plots outside of the analysed epoch (3-bin boxcar for the inference trial on single-units), and either a 3-bin boxcar (for Fig. 2 ) or no smoothing ( Fig. 3 ) being used within the analysed epoch. For population average activity displays ( Figs 4 , 5 and 7 ), a 5-bin boxcar was used. To make plots of trial-by-trial choice rate, we first aligned all rewarded trials for all blocks, and for each trial (1st, 2nd, 3rd and so on after the block switch), we took the proportion of choices towards the side with the three-drop reward, excluding all blocks in which a forced-choice trial happened to occur on that trial. For Fig. 1 , line was then smoothed using a 3-bin boxcar, separately for before and after the switch. How to cite this article: Stalnaker, T. A. et al . Orbitofrontal neurons infer the value and identity of predicted outcomes. Nat. Commun. 5:3926 doi: 10.1038/ncomms4926 (2014). The opinions expressed in this article are the authors' own and do not reflect the view of the National Institutes of Health, the Department of Health and Human Services, or the United States government.